MafB promotes atherosclerosis by inhibiting foam-cell apoptosis MafB is a transcription factor that induces myelomonocytic differentiation. However, the precise role of MafB in the pathogenic function of macrophages has never been clarified. Here we demonstrate that MafB promotes hyperlipidemic atherosclerosis by suppressing foam-cell apoptosis. Our data show that MafB is predominantly expressed in foam cells found within atherosclerotic lesions, where MafB mediates the oxidized LDL-activated LXR/RXR-induced expression of apoptosis inhibitor of macrophages (AIM). In the absence of MafB, activated LXR/RXR fails to induce the expression of AIM, a protein that is normally responsible for protecting macrophages from apoptosis; thus, Mafb -deficient macrophages are prone to apoptosis. Haematopoietic reconstitution with Mafb -deficient fetal liver cells in recipient LDL receptor-deficient hyperlipidemic mice revealed accelerated foam-cell apoptosis, which subsequently led to the attenuation of the early atherogenic lesion. These findings represent the first evidence that the macrophage-affiliated MafB transcription factor participates in the acceleration of atherogenesis. Macrophages are essential in the development of atherosclerosis [1] , [2] , [3] . In the early stages of atherosclerosis, accumulation of highly oxidized low-density lipoprotein (oxLDL) in the intima induces dysfunction of endothelial cells and smooth muscle cells (SMCs), leading to the production of proinflammatory cytokines including chemokines that recruit monocytes. These recruited monocytes become macrophages that take up oxLDL via scavenger receptors. Then, the pathogenic macrophages transform into foam cells and form the fatty streak, which constitutes the early atherogenic lesion and eventually gives rise to the more advanced atheromatous plaques. Accumulation of toxic oxLDL induces apoptosis in a variety of cell types, including macrophages; therefore, the foam cells found in atherogenic lesions are inclined to undergo apoptosis [4] . However, pathological aberrations in foam cells have been shown to exacerbate atherogenesis. For instance, a deficiency of pro-apoptotic factors, such as Bax and p53, suppresses the apoptosis of foam cells and thereby accelerates atherosclerosis progression [5] , [6] . On the other hand, the increased apoptosis of foam cells induced by the disruption of EP4 (the PGE2 receptor) reduces the size of early atherogenic lesions [7] . These observations support the concept that the accelerated apoptosis of foam cells could lead to reduced lesion size and a subsequent attenuation of plaque progression [5] , [7] , [8] , [9] , [10] , [11] . The gene product of the c- Maf proto-oncogene and its relatives (the large Maf family of transcription factors) share conserved basic regions and an amphipathic helix (bZIP) domain that mediate their binding to Maf recognition elements (MAREs [12] ) and their dimerization, respectively. Each of the large Maf proteins (MafA/L-Maf/SMaf, MafB, c-Maf and Nrl) contains an acidic domain that promotes transcriptional activation and plays crucial roles in cellular differentiation in various tissues [12] , [13] , [14] , [15] , [16] , [17] , [18] , [19] , [20] . In haematopoietic lineages, MafB is expressed selectively in monocytes and macrophages but not in other mature myeloid or lymphoid lineages [18] , [21] , [22] . In vitro studies have demonstrated that MafB induces myelomonocytic differentiation in immortalized myeloblasts and human CD34 + haematopoietic stem cells [18] , [23] , [24] , [25] . However, Mafb -deficient embryos retain a normal population of Mac-1-positive myeloid cells, although these cells fail to express the F4/80 marker for differentiated resident macrophages [26] . Another group reported that the increased expression of actin-organizing factors in Mafb -deficient macrophages leads to morphological abnormalities in macrophages [27] . Together, these analyses suggest multiple roles for MafB in the terminal macrophage maturation stage. Meanwhile, several lines of evidence have recently emerged suggesting a relationship between MafB and atherosclerosis. Gene expression profiling of bone marrow macrophages from apoE -deficient atherosclerotic mice with several genetic backgrounds showed that MafB is most abundantly expressed in the macrophages of mice with a more susceptible genetic background [28] . A human genome-wide analysis showed that the MAFB locus is close to a susceptibility single-nucleotide polymorphism that is associated with high levels of serum LDL cholesterol [29] . These observations imply that MafB might play a pathogenic role in the development of atherosclerotic lesions. Moreover, MafB expressed in alveolar macrophages participates in the pathophysiology of chronic obstructive pulmonary disease that is related to cigarette smoking [30] . AIM (AIM/Api6/Spα) is a member of the scavenger receptor cysteine-rich superfamily and exerts an anti-apoptotic function in macrophages [31] , [32] , [33] . Disruption of AIM expression can decrease the development of early atherosclerotic lesions by increasing the apoptotic cell death of foam cells [8] . AIM expression is induced by the heterodimerized nuclear receptor liver X receptor (LXR)/retinoid X receptor (RXR), which is activated upon the accumulation of oxLDL in mature tissue macrophages [8] , [33] , [34] . In the present study, we demonstrate that MafB is expressed in the foam cells and enhances their survival in aortic atherosclerotic lesions. MafB deficiency in the foam cells led to accelerated apoptosis due to reduced AIM expression and consequently ameliorated atherosclerotic lesions in LDL receptor-deficient ( LDLR −/− ) hyperlipidemic mice. MafB expression in the foam cells of atherosclerotic lesions To examine the distribution of MafB-expressing macrophages within atherosclerotic lesions, immunofluorescence analysis was performed on atherosclerotic plaques, which developed in the aortic roots of LDLR −/− mice fed an atherogenic diet for 8 weeks [35] . The atherosclerotic plaques in the LDLR −/− mice harboured numerous lipid-filled foam cells, which were visualized by Oil Red O staining and cell surface Mac-2 and nuclear MafB expression ( Fig. 1a–f ). Of note, the majority of MafB-positive cells colocalized with Mac-2-positive signals and Hoechst ( Fig. 1g–j ). 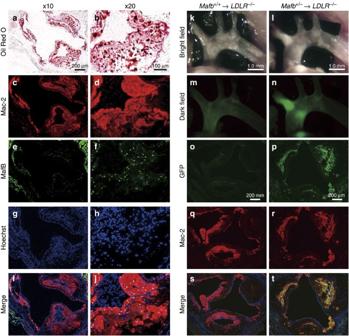Figure 1: MafB is expressed in foam cells found within atherosclerotic lesions ofLDLR−/−mice. (a–j) Atherosclerotic lesions around the aortic root ofLDLR−/−mice fed an atherogenic diet for 8 weeks were subjected to immunohistochemical analyses. Serial adjacent sections were stained with Oil Red O, anti-Mac-2 (macrophage marker, red), anti-MafB (green) and Hoechst (blue). Left and right columns show lower (a,c,e,g,i; scale bar, 200 μm) and higher magnification images (b,d,f,h,j; scale bar, 100 μm), respectively. (l,n) Stereoscopic observations show GFP fluorescence in atheromatous plaques around the aortic arch inMafb+/−→LDLR−/−mice. (k,m) TheMafb+/+→LDLR−/−control mouse exhibited no GFP fluorescence. Expression of GFP (o,p, green) and Mac-2 (q,r, red) in atherosclerotic lesions ofMafb+/+→LDLR−/−orMafb+/−→LDLR−/−mice were analyzed by immunohistochemistry. (s,t) TheMafb+/−→LDLR−/−mouse exhibited GFP immunoreactivity in Mac-2 positive area. Figure 1: MafB is expressed in foam cells found within atherosclerotic lesions of LDLR −/− mice. ( a – j ) Atherosclerotic lesions around the aortic root of LDLR −/− mice fed an atherogenic diet for 8 weeks were subjected to immunohistochemical analyses. Serial adjacent sections were stained with Oil Red O, anti-Mac-2 (macrophage marker, red), anti-MafB (green) and Hoechst (blue). Left and right columns show lower ( a , c , e , g , i ; scale bar, 200 μm) and higher magnification images ( b , d , f , h , j ; scale bar, 100 μm), respectively. ( l , n ) Stereoscopic observations show GFP fluorescence in atheromatous plaques around the aortic arch in Mafb +/− → LDLR −/− mice. ( k , m ) The Mafb +/+ → LDLR −/− control mouse exhibited no GFP fluorescence. Expression of GFP ( o , p , green) and Mac-2 ( q , r , red) in atherosclerotic lesions of Mafb +/+ → LDLR −/− or Mafb +/− → LDLR −/− mice were analyzed by immunohistochemistry. ( s , t ) The Mafb +/− → LDLR −/− mouse exhibited GFP immunoreactivity in Mac-2 positive area. Full size image Previously, we demonstrated that GFP expression in the Mafb -GFP knock-in ( Mafb − allele) mouse faithfully recapitulates endogenous MafB expression [26] . To clarify the involvement of the GFP-positive MafB-expressing cells in the atherosclerotic lesions, we examined GFP expression in lethally irradiated LDLR −/− mice reconstituted with the embryonic day (E) 14.5 Mafb +/− fetal liver haematopoietic cells. After an 8-week recovery period, the LDLR −/− recipient mice were fed an atherosclerosis-inducing diet for the next 5 weeks. GFP fluorescence was clearly observed in the aortic arch of the LDLR −/− mice that received the Mafb +/− fetal liver cells ( Mafb +/− → LDLR −/− ) but not in those transplanted with the Mafb +/+ fetal liver cells ( Mafb +/+ → LDLR −/− ) ( Fig. 1k–n ). Immunohistochemical analysis using anti-GFP and Mac-2 antibodies showed that the GFP-positive cells were coincident with the Mac-2-positive lipid-filled foam cells ( Fig. 1p,r,t ). In contrast, GFP-positive cells were not observed in the Mafb +/+ → LDLR −/− recipients, as expected ( Fig. 1o,q,s ). These results clearly indicate that MafB is expressed in the foam cells found within the atherosclerotic lesions of hyperlipidemic LDLR −/− mice, implying a functional role for MafB in atherogenesis. Suppression of atherogenesis in the Mafb -deficient mice To investigate the functional role of haematopoietic MafB expression in atherogenesis, the haematopoietic system of lethally irradiated LDLR −/− mice was reconstituted with the transplantation of E14.5 fetal liver cells prepared from Mafb +/+ and Mafb −/− embryos. MafB expression was virtually absent in the diet-induced atherosclerotic lesions of LDLR −/− mice transplanted with Mafb −/− fetal liver cells ( Mafb −/− → LDLR −/− ) ( Supplementary Fig. 1a ). To our surprise, the development of atherosclerotic lesions was dramatically decreased in the Mafb −/− → LDLR −/− recipient mice in comparison with the Mafb +/+ → LDLR −/− mice ( Fig. 2a,b,d,e ) after the animals were fed an atherogenic diet for 5 weeks or 12 weeks. Quantification of the area covered by the atherosclerotic lesion around the aortic valve revealed a statistically significant decrease in lesion size in the Mafb −/− → LDLR −/− recipient mice, regardless of gender ( Fig. 2c,f ). An en face preparation along the entire aorta also showed a stark contrast between the Mafb −/− → LDLR −/− and Mafb +/+ → LDLR −/− recipient mice with regard to the expansion of Oil Red O-positive atheromatous plaques after 5 weeks or 12 weeks of an atherogenic diet ( Fig. 2g,h,j,k ). Quantification of the atherosclerotic lesion area of the en face preparation showed a consistent decrease when MafB was absent in the haematopoietic system ( Fig. 2i,l ). Moreover, we performed Masson’s trichrome staining and immunohistochemistry analysis using anti-CD31 (endothelial cells), anti-α-actin (SMCs) and anti-CD3 (T cells). Although the total areas of collagen, SMCs and T cells were also decreased due to less advanced lesions in Mafb −/− → LDLR −/− , some of them were not significantly different per unit area ( Supplementary Fig. 2 ). We observed no significant differences in either body weight or plasma cholesterol between the Mafb +/+ → LDLR −/− and Mafb −/− → LDLR −/− mice after the consumption of a high-cholesterol diet for 5, 8 or 10 weeks, indicating that MafB deficiency does not have a major impact on lipid metabolism ( Table 1 ). Furthermore, haematological analysis of peripheral blood showed no differences between genotypes ( Supplementary Fig. 3a ). Additionally, there were no significant differences in the number of B220-, CD4-/8- or Mac-1-positive cells in peripheral blood, spleen or bone marrow by flow cytometry analysis ( Supplementary Fig. 3b ). Overall, these haematopoietic reconstitution analyses demonstrate that haematopoietic MafB is a key exacerbating factor in the progression of atherosclerosis. 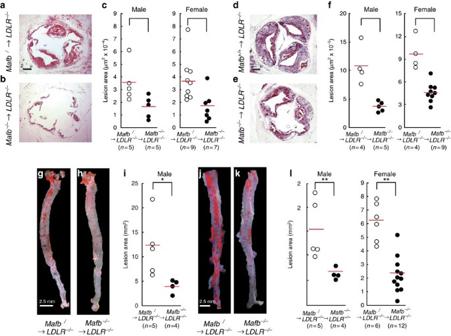Figure 2: Reduction of atherogenic lesions inMafb−/−→LDLR−/−mice. (a–f) Frozen sections from the aortic roots ofMafb+/+→LDLR−/−andMafb−/−→LDLR−/−mice fed an atherogenic diet for 5 weeks (a,b) or 12 weeks (d,e) were stained with Oil Red O. The surface area of the Oil Red O-positive atherosclerotic lesions of both male and female mice after treatment with an atherogenic diet for 5 weeks (c) or 12 weeks (f) were quantified. Each symbol in the scatter plots represents the lesion area of one independent mouse. The horizontal bar indicates the mean lesion size. (g–l) Representative photographs fromen faceanalysis of aortas fromMafb+/+→LDLR−/−andMafb−/−→LDLR−/−recipient mice after 5 weeks (g,h) or 12 weeks (j,k) on a high-cholesterol diet. The surface area of the Oil Red O-positive atherosclerotic lesions from theen facepreparation after treatment with atherogenic diet for 5 weeks (i) or 12 weeks (l) was quantified. Each symbol in the scatter plots represents the lesion area of one independent mouse. The horizontal bar indicates mean lesion size. *P<0.05, **P<0.01 (Student’st-test). Figure 2: Reduction of atherogenic lesions in Mafb −/− → LDLR −/− mice. ( a – f ) Frozen sections from the aortic roots of Mafb +/+ → LDLR −/− and Mafb −/− → LDLR −/− mice fed an atherogenic diet for 5 weeks ( a , b ) or 12 weeks ( d , e ) were stained with Oil Red O. The surface area of the Oil Red O-positive atherosclerotic lesions of both male and female mice after treatment with an atherogenic diet for 5 weeks ( c ) or 12 weeks ( f ) were quantified. Each symbol in the scatter plots represents the lesion area of one independent mouse. The horizontal bar indicates the mean lesion size. ( g – l ) Representative photographs from en face analysis of aortas from Mafb +/+ → LDLR −/− and Mafb −/− → LDLR −/− recipient mice after 5 weeks ( g , h ) or 12 weeks ( j , k ) on a high-cholesterol diet. The surface area of the Oil Red O-positive atherosclerotic lesions from the en face preparation after treatment with atherogenic diet for 5 weeks ( i ) or 12 weeks ( l ) was quantified. Each symbol in the scatter plots represents the lesion area of one independent mouse. The horizontal bar indicates mean lesion size. * P< 0.05, ** P< 0.01 (Student’s t -test). Full size image Table 1 Plasma lipid levels in LDLR −/− mice transplanted with Mafb +/+ or Mafb −/− fetal liver cells. Full size table Reduced expression of AIM in Mafb −/− macrophages As MafB is predominantly expressed in the macrophages of the haematopoietic system [22] , [26] , we hypothesized that the attenuation of atherogenic lesions in the Mafb −/− → LDLR −/− mice could be attributed to functional alterations in the Mafb −/− macrophages. To comprehensively examine the gene expression profile of the Mafb -deficient macrophages, we performed gene expression microarray analysis using M-CSF-induced fetal liver-derived macrophages [26] . The most drastic expression change observed in the expression microarray analysis was a 90% reduction of AIM expression in the Mafb −/− fetal liver macrophages. Consistently, AIM mRNA was reproducibly diminished to 20% of the Mafb +/+ level in the Mafb −/− fetal liver macrophages, as determined by real-time quantitative reverse transcription PCR (qRT–PCR) analysis ( Fig. 3a , left panel). Antiserum raised against the AIM protein was used to detect basal AIM protein expression by immunocytochemistry in the cultured Mafb +/+ fetal liver-derived macrophages ( Fig. 3b ). LXR/RXR activation, which was induced by treatment with a combination of T0901317 (T1317, a synthetic agonist of LXR) and 9- cis -retinoic acid (9cRA, a ligand for RXR), increased the AIM mRNA expression up to 20-fold in the Mafb +/+ fetal liver macrophages. In contrast, T1317/9cRA administration barely induced AIM expression in the Mafb −/− fetal liver macrophages ( Fig. 3a , right panel). In agreement with this observation, the T1317/9cRA treatment increased the AIM staining intensity of the Mafb +/+ fetal liver macrophages ( Fig. 3b,c ). However, AIM immunoreactivity was barely detectable in the Mafb −/− fetal liver-derived macrophages, regardless of T1317/9cRA treatment ( Fig. 3b,c ). These data indicate that MafB mediates activated LXR/RXR-induced AIM expression in primary fetal liver macrophages. 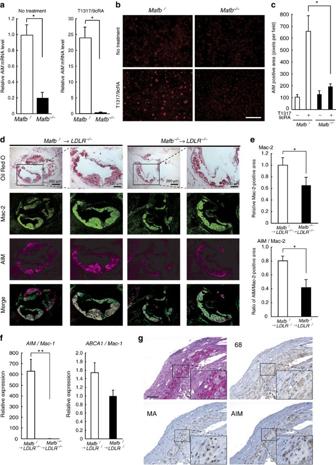Figure 3: AIM expression is reduced inMafb-deficient macrophages. (a) TheAIMmRNA levels inMafb+/+andMafb−/−fetal liver-derived macrophages were examined by qRT–PCR (Mafb+/+,n=6;Mafb−/−,n=6). Data were normalized to theHprtmRNA and are presented as the mean+s.e.m. *P<0.05 (Student’st-test). (b) Immunocytochemical analysis of AIM protein expression inMafb+/+andMafb−/−fetal liver-derived macrophages. The cells were stained with anti-AIM antibody. (a,b) The macrophages were incubated for 24 h with or without a mixture of T1317 (LXR agonist, 1 μM) and 9cRA (RXR agonist, 1 μM). (c) The AIM-positive area of the field of confluent cells was morphometrically quantified. Data are presented as the mean+s.e.m. Ten fetal liver-derived macrophages (Mafb+/+,n=4;Mafb−/−,n=6) were analyzed. *P<0.05 (Student’st-test) (d) Serial sections of 5-week diet-induced atheromatous plaques inLDLR−/−recipient mice were stained with Oil Red O, anti-Mac-2 and anti-AIM. (e) The Mac-2-positive area (upper panel) and the AIM-positive area relative to the Mac-2-positive area (AIM/Mac-2 ratio; lower panel) in the atherosclerotic lesions were morphometrically quantified. Data are presented as the mean+s.e.m. Thirteen mice (Mafb+/+,n=8;Mafb−/−,n=5) were analyzed. *P<0.05 (Student’st-test). (f) The qRT–PCR showed the expression ofAIMandABCA1mRNA in the atherosclerotic lesions ofMafb+/+→LDLR−/−andMafb−/−→LDLR−/−recipient mice after 5 weeks of a high-cholesterol diet (Mafb+/+,n=8;Mafb−/−,n=8). Data are presented as the mean+s.e.m. **P<0.01 (Student’st-test). (g) Serial adjacent sections of a human atherosclerotic lesion were stained with haematoxylin–eosin, anti-CD68 (macrophage marker), anti-MAFB and anti-AIM. Signals of CD68, MAFB and AIM were observed in the same region. Similar results were obtained in the three types of specimens. Scale bar, 100 μm. Figure 3: AIM expression is reduced in Mafb -deficient macrophages. ( a ) The AIM mRNA levels in Mafb +/+ and Mafb −/− fetal liver-derived macrophages were examined by qRT–PCR ( Mafb +/+ , n =6; Mafb −/− , n =6). Data were normalized to the Hprt mRNA and are presented as the mean+s.e.m. * P< 0.05 (Student’s t -test). ( b ) Immunocytochemical analysis of AIM protein expression in Mafb +/+ and Mafb −/− fetal liver-derived macrophages. The cells were stained with anti-AIM antibody. ( a , b ) The macrophages were incubated for 24 h with or without a mixture of T1317 (LXR agonist, 1 μM) and 9cRA (RXR agonist, 1 μM). ( c ) The AIM-positive area of the field of confluent cells was morphometrically quantified. Data are presented as the mean+s.e.m. Ten fetal liver-derived macrophages ( Mafb +/+ , n =4; Mafb −/− , n =6) were analyzed. * P< 0.05 (Student’s t -test) ( d ) Serial sections of 5-week diet-induced atheromatous plaques in LDLR −/− recipient mice were stained with Oil Red O, anti-Mac-2 and anti-AIM. ( e ) The Mac-2-positive area (upper panel) and the AIM-positive area relative to the Mac-2-positive area (AIM/Mac-2 ratio; lower panel) in the atherosclerotic lesions were morphometrically quantified. Data are presented as the mean+s.e.m. Thirteen mice ( Mafb +/+ , n =8; Mafb −/− , n =5) were analyzed. * P< 0.05 (Student’s t -test). ( f ) The qRT–PCR showed the expression of AIM and ABCA1 mRNA in the atherosclerotic lesions of Mafb +/+ → LDLR −/− and Mafb −/− → LDLR −/− recipient mice after 5 weeks of a high-cholesterol diet ( Mafb +/+ , n =8; Mafb −/− , n =8). Data are presented as the mean+s.e.m. ** P< 0.01 (Student’s t -test). ( g ) Serial adjacent sections of a human atherosclerotic lesion were stained with haematoxylin–eosin, anti-CD68 (macrophage marker), anti-MAFB and anti-AIM. Signals of CD68, MAFB and AIM were observed in the same region. Similar results were obtained in the three types of specimens. Scale bar, 100 μm. Full size image To clarify whether AIM expression is dependent on MafB in the foam cells of atherosclerotic lesions, we performed immunofluorescence analysis with the anti-AIM antibody ( Fig. 3d and Supplementary Fig. 1b ). Consistent with the qRT–PCR analysis, the AIM staining intensity was diminished in the atherosclerotic lesions of the Mafb −/− → LDLR −/− recipient mice compared with the Mafb +/+ → LDLR −/− mice ( Fig. 3d ). To quantify the AIM immunoreactivity, the AIM-positive surface area and Mac-2-positive surface area in the atherosclerotic lesions were morphometrically analyzed. Of note, the Mac-2-positive foam-cell area was smaller in the Mafb −/− → LDLR −/− recipients than in the Mafb +/+ → LDLR −/− mice, confirming the reduced size of the atherosclerotic lesions in the Mafb −/− → LDLR −/− mice ( Fig. 3d,e , upper panel). Furthermore, the ratio of the AIM-positive surface area to the Mac-2-positive surface area (AIM/Mac-2 ratio) was also significantly lower in the Mafb −/− → LDLR −/− mice than in the Mafb +/+ → LDLR −/− mice ( Fig. 3e , lower panel). Moreover, we cut the aorta in the atherosclerotic lesion with a small pair of scissors. The small pieces of aorta including the atherosclerotic lesion were analyzed by qRT–PCR. The results showed that a >600-fold reduction of AIM mRNA occurred in the Mafb −/− → LDLR −/− mice compared with the Mafb +/+ → LDLR −/− mice, while the ABCA1 expression level was not significantly different ( Fig. 3f ). We also examined the expression of MAFB and AIM in human atherosclerotic lesions (human thoracic aorta). An immunohistochemical analysis showed that the signal of anti-AIM and MAFB was detected in the CD68-positive macrophage area in human atherosclerotic lesions ( Fig. 3g ). This result suggests that in human atherosclerotic lesions, MAFB may regulate the expression of AIM. These observations strongly suggest that MafB is crucial for hyperlipidemia-induced AIM expression in the foam cells of atherosclerotic lesions. Among the four large mammalian Maf transcription factors, MafB and c-Maf are expressed in the monocyte–macrophage lineage [36] , [37] . Notably, c-Maf -deficient fetal liver-derived macrophages maintained T1317/9cRA-induced AIM expression, indicating that MafB is more important than c-Maf for LXR/RXR-induced AIM expression in macrophages ( Supplementary Fig. 4a ). MafB is essential for the inhibition of foam-cell apoptosis AIM deficiency accelerates oxLDL-induced apoptosis in cultured macrophages. AIM -deficient mice exhibit increased apoptosis in the foam cells of atherosclerotic lesions [8] . These data prompted us to examine whether the reduced AIM expression in Mafb -deficient macrophages promotes increased apoptosis in atherosclerotic lesions. oxLDL-induced apoptosis in the Mafb +/+ and Mafb −/− macrophages was quantitatively assessed by an activity assay for cleaved caspase-3. As anticipated, the activity of cleaved caspase-3, measured by a homogeneous luminescent assay, was increased in the Mafb −/− macrophages compared with the Mafb +/+ macrophages upon oxLDL treatment (50 and 100 μg ml −1 ; Fig. 4a,b ). Terminal deoxynucleotidyl transferase-mediated dUTP nick-end labelling (TUNEL) analysis of atherosclerotic lesions after mice were fed an atherogenic diet for 5 and 12 weeks revealed that apoptotic cells were increased in the Mafb −/− → LDLR −/− mice compared with the Mafb +/+ → LDLR −/− control mice ( Fig. 4c,d ). Moreover, immunostaining of the atherosclerotic lesions with an anti-cleaved caspase-3 antibody showed that the cleaved caspase-3-positive population was significantly increased in the Mafb −/− → LDLR −/− mice compared with the Mafb +/+ → LDLR −/− control mice after 7–8 or 12 weeks on a high-cholesterol diet ( Fig. 4e,f ). To confirm whether cleaved caspase-3-positive cells were macrophages or other cells, we performed multicolor fluorescence immunostaining using anti-cleaved caspase-3 antibody and anti-Mac-2 antibody. As expected, cleaved caspase-3-positive cells also expressed Mac-2 ( Supplementary Fig. 5 ). These results suggested that macrophage apoptosis in Mafb −/− was increased in the oxLDL-treated cultures as well as in hyperlipidemic condition of LDLR -deficient mice. 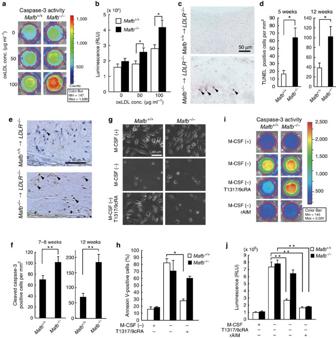Figure 4: Apoptosis is accelerated inMafb−/−macrophages due to reduced AIM expression. (a) Luminescence assays were performed to measure cleaved caspase-3 activity. Representative luminescent signals are shown forMafb+/+andMafb−/−macrophages incubated with various concentrations of oxLDL for 16 h. (b) Quantification of luminescence intensity (RLU, relative light units).Mafb+/+,n=7;Mafb−/−,n=6. (c) TUNEL staining of atherosclerotic lesions fromMafb+/+→LDLR−/−andMafb−/−→LDLR−/−mice fed an atherogenic diet for 12 weeks. (d) The number of TUNEL-positive cells per mm2was quantified at 5 weeks and 12 weeks (Mafb+/+, n=4;Mafb−/−, n=4). (e) Cleaved caspase-3 staining of atherosclerotic lesions fromMafb+/+→LDLR−/−andMafb−/−→LDLR−/−mice fed an atherogenic diet for 12 weeks (c,e; scale bar, 50 μm). (f) The number of cleaved caspase-3-positive cells per mm2was quantified at 7–8 weeks (Mafb+/+,n=9;Mafb−/−,n=8) and 12 weeks (Mafb+/+,n=4;Mafb−/−,n=4). (g–j) fetal liver-derived macrophages were prestimulated with a combination of T1317 (LXR agonist, 1 μM) and 9cRA (RXR agonist, 1 μM) for 17–24 h or with recombinant AIM (rAIM, 50 μg ml−1) for 3 h. Apoptosis was induced by the withdrawal of M-CSF for 24 h (g) or 10 h (i). LXR/RXR agonists and rAIM were added to the M-CSF-free media. (g) Bright-field images depict apoptotic cell death and restoration upon agonist treatment (scale bar, 50 μm). (h) The percentage of Annexin V-positive apoptotic macrophages was quantified by flow cytometry.Mafb+/+,n=3;Mafb−/−,n=3. Note the significant improvement in the agonist-treatedMafb−/−macrophages. (i) Cleaved caspase-3 activity of representative luminescent signals was measured as described above. (j) Quantification of luminescence intensity.Mafb+/+,n=6;Mafb−/−,n=6. (b,d,f,h,j) Quantification data are presented as the mean+s.e.m. *P<0.05, **P<0.01 (Student’st-test). Figure 4: Apoptosis is accelerated in Mafb −/− macrophages due to reduced AIM expression. ( a ) Luminescence assays were performed to measure cleaved caspase-3 activity. Representative luminescent signals are shown for Mafb +/+ and Mafb −/− macrophages incubated with various concentrations of oxLDL for 16 h. ( b ) Quantification of luminescence intensity (RLU, relative light units). Mafb +/+ , n =7; Mafb −/− , n =6. ( c ) TUNEL staining of atherosclerotic lesions from Mafb +/+ → LDLR −/− and Mafb −/− → LDLR −/− mice fed an atherogenic diet for 12 weeks. ( d ) The number of TUNEL-positive cells per mm 2 was quantified at 5 weeks and 12 weeks ( Mafb +/+ , n=4; Mafb −/− , n=4). ( e ) Cleaved caspase-3 staining of atherosclerotic lesions from Mafb +/+ → LDLR −/− and Mafb −/− → LDLR −/− mice fed an atherogenic diet for 12 weeks ( c , e ; scale bar, 50 μm). ( f ) The number of cleaved caspase-3-positive cells per mm 2 was quantified at 7–8 weeks ( Mafb +/+ , n =9; Mafb −/− , n =8) and 12 weeks ( Mafb +/+ , n =4; Mafb −/− , n =4). ( g – j ) fetal liver-derived macrophages were prestimulated with a combination of T1317 (LXR agonist, 1 μM) and 9cRA (RXR agonist, 1 μM) for 17–24 h or with recombinant AIM (rAIM, 50 μg ml −1 ) for 3 h. Apoptosis was induced by the withdrawal of M-CSF for 24 h ( g ) or 10 h ( i ). LXR/RXR agonists and rAIM were added to the M-CSF-free media. ( g ) Bright-field images depict apoptotic cell death and restoration upon agonist treatment (scale bar, 50 μm). ( h ) The percentage of Annexin V-positive apoptotic macrophages was quantified by flow cytometry. Mafb +/+ , n =3; Mafb −/− , n =3. Note the significant improvement in the agonist-treated Mafb −/− macrophages. ( i ) Cleaved caspase-3 activity of representative luminescent signals was measured as described above. ( j ) Quantification of luminescence intensity. Mafb +/+ , n =6; Mafb −/− , n =6. ( b , d , f , h , j ) Quantification data are presented as the mean+s.e.m. * P< 0.05, ** P< 0.01 (Student’s t -test). Full size image Apoptosis of macrophages can be induced by various stimuli, such as oxLDL, cytokine depletion, cycloheximide or bacteria, but is inhibited by treatment with agonists of LXR and RXR. Furthermore, small interfering RNA (siRNA) knockdown of AIM attenuates the apoptosis-inhibitory effects exerted by LXR/RXR agonist treatment, suggesting that AIM is required for the efficacy of LXR/RXR agonists [33] . Given the crucial role that MafB plays in AIM induction following LXR/RXR activation, we assumed that the apoptosis-inhibitory effect of LXR/RXR agonist treatment depends on MafB. To address this hypothesis, we examined the effect of MafB deficiency on the anti-apoptotic efficacy of the LXR/RXR agonists. Cytokine depletion-induced apoptosis in the wild-type macrophages, which was quantified by the number of annexin V-positive cells and the activity of cleaved caspase-3, was significantly attenuated by the administration of T1317/9cRA ( Fig. 4g–j ). However, the induced apoptosis of the Mafb −/− macrophages was not rescued by T1317/9cRA treatment. Administration of recombinant AIM inhibited the apoptosis of Mafb −/− macrophages, indicating that the Mafb −/− macrophages were still responsive to the AIM-mediated anti-apoptotic effect ( Fig. 4i,j ). Taken together, these results underscore the prime importance of MafB in the inhibition of macrophage apoptosis, as it mediates the LXR/RXR–AIM regulatory axis. In fact, expression levels of both Mafb and AIM were significantly increased in macrophages treated with oxLDL ( Supplementary Fig. 6a ). Moreover, qRT–PCR using mRNA obtained from atherosclerotic lesions indicated that Mafb and AIM were highly increased compared with their levels in control macrophages ( Supplementary Fig. 6b ). These results indicate that MafB and AIM expression are synchronously induced in the hyperlipidaemic condition. As the migration of macrophages underneath the vascular endothelium is essential for the initiation of atherogenesis, we next examined the motility potential of the Mafb -deficient macrophages. The number of peritoneal macrophages recruited by thioglycolate administration barely differed between the Mafb +/+ → LDLR −/− and Mafb −/− → LDLR −/− recipient mice ( Supplementary Fig. 7a ). The mRNA abundance of macrophage chemoattractant protein-1 (MCP-1), a crucial attractant for macrophage migration, also barely differed between the two genotypes ( Supplementary Fig. 7b ). Moreover, IL-6, IL-12p40 and IL-10 production were not significantly different between Mafb +/+ and Mafb −/− macrophages ( Supplementary Fig. 8 ). The T1317/9cRA-induced mRNA expression of ABCA1 (ATP-binding cassette A1) and ABCG1 (ATP-binding cassette G1), two representative ATP-binding cassette transporters for cholesterol efflux, were equally increased in both genotypes of fetal liver macrophages, indicating that cholesterol extractability was not altered in the Mafb -deficient macrophages ( Supplementary Fig. 9b,c ). We also examined oxLDL and acLDL uptake in the Mafb -deficient macrophages. Upon treatment with DiI-oxLDL or DiI-acLDL for 24 h, no significant differences were observed between Mafb +/+ and Mafb −/− macrophages by fluorescence-activated cell sorting (FACS) analysis ( Supplementary Fig. 10 ). Overall, these results confirm that MafB deficiency does not significantly affect the number or basic function of macrophages. MafB directly regulates AIM gene expression Next, to determine whether MafB directly regulates AIM expression, we searched for putative transcription factor-binding sites in the promoter of the AIM gene using the UCSC Genome Browser ( http://genome.ucsc.edu/index.html ). Of note, a potential MARE site was identified −54 bp upstream of the transcription initiation site that is highly conserved among multiple mammalian species ( Fig. 5a ). A series of luciferase reporter constructs were tested by co-transfection with a MafB expression vector in the H441 cell line. The −1993/Luc and the −473/Luc reporter constructs, both of which contained a proximal MARE site, were significantly activated by the co-introduction of MafB in a plasmid dose-dependent manner ( Fig. 5b ). Expectedly, the −34/Luc deletion mutants and the mutant with a substitution in the conserved MARE site (−473+mut/Luc) showed dramatically diminished responsiveness to MafB co-expression ( Fig. 5b ). Electrophoretic mobility shift assays (EMSAs) demonstrated that a double-stranded DNA oligonucleotide containing the MARE site was specifically bound by MafB proteins expressed in 293 T cells ( Fig. 5c ). As expected, the mutant oligonucleotides failed to competitively inhibit MARE-specific MafB binding ( Fig. 5c , lane 5). To confirm direct MafB binding and subsequent changes in the epigenetic mark at the MARE site, we conducted a chromatin immunoprecipitation (ChIP) assay using anti-MafB and anti-acetylated H4 (AcH4) antibodies in fetal liver macrophages. T1317/9cRA treatment significantly increased AcH4 and MafB occupancy at the MARE sites of the AIM promoter region ( Fig. 5d ). This observation indicates that MafB directly binds to the MARE site and activates AIM gene expression upon LXR/RXR agonist treatment. Taken together, these data demonstrate that MafB regulates AIM gene expression by directly binding to the highly conserved MARE element in the promoter region. 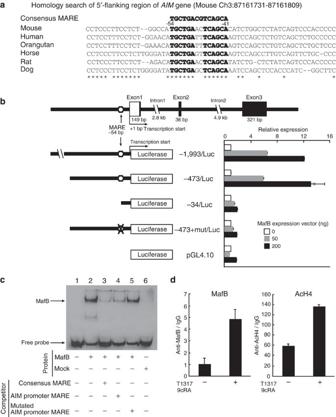Figure 5: Identification of MafB-responsive regions in theAIMpromoter. (a) The 5′-flanking region of theAIMgene was analyzed with the UCSC Genome Browser to identify MafB-binding sites (Maf Recognition Element; MARE). The MARE site in theAIMpromoter (mouse: −54/−41, bold) is highly conserved among mammalian species. (b) A co-transfection reporter assay was performed in the H441 cell line using vectors expressing a series ofAIMpromoter deletion mutants and a MafB expression vector. The relative luciferase activities of the reporter constructs induced by the co-expression of MafB are shown on the right and are presented as fold values relative to the basal activity. The term ‘mut’ denotes a substitution mutation in the MARE site (seeMethods). Data are from one experiment representative of three independent experiments and presented as mean+s.e.m. of duplicate. (c) EMSA with a probe for the MARE site in theAIMpromoter. MafB and mock-control proteins were prepared by transfecting 293 T cells with MafB and mock expression vectors. The consensus MARE sequences were described previously12. (d) Chromatin from the pool of fetal liver macrophages (WT,n=6) with or without agonist treatment (T1317 and 9cRA) was precipitated with anti-MafB, anti-AcH4 and IgG and then analyzed by qPCR to amplify the MARE sequences in theAIMpromoter region. The s.d. was representative of the variation in the technical triplicates of samples. Data are from one experiment representative of two independent experiments. Figure 5: Identification of MafB-responsive regions in the AIM promoter. ( a ) The 5′-flanking region of the AIM gene was analyzed with the UCSC Genome Browser to identify MafB-binding sites (Maf Recognition Element; MARE). The MARE site in the AIM promoter (mouse: −54/−41, bold) is highly conserved among mammalian species. ( b ) A co-transfection reporter assay was performed in the H441 cell line using vectors expressing a series of AIM promoter deletion mutants and a MafB expression vector. The relative luciferase activities of the reporter constructs induced by the co-expression of MafB are shown on the right and are presented as fold values relative to the basal activity. The term ‘mut’ denotes a substitution mutation in the MARE site (see Methods ). Data are from one experiment representative of three independent experiments and presented as mean+s.e.m. of duplicate. ( c ) EMSA with a probe for the MARE site in the AIM promoter. MafB and mock-control proteins were prepared by transfecting 293 T cells with MafB and mock expression vectors. The consensus MARE sequences were described previously [12] . ( d ) Chromatin from the pool of fetal liver macrophages (WT, n =6) with or without agonist treatment (T1317 and 9cRA) was precipitated with anti-MafB, anti-AcH4 and IgG and then analyzed by qPCR to amplify the MARE sequences in the AIM promoter region. The s.d. was representative of the variation in the technical triplicates of samples. Data are from one experiment representative of two independent experiments. Full size image MafB expression is activated by LXR/RXR in macrophages Assuming a potential genetic hierarchy between LXR/RXR, MafB and AIM, we next examined whether agonist-activated LXR/RXR induces MafB expression in fetal liver-derived macrophages. T1317/9cRA administration sharply induced Mafb mRNA expression, up to 4.5-fold in 2 h in wild-type fetal liver macrophages ( Fig. 6a ). This Mafb induction was associated with a gradual increase in AIM mRNA abundance (a maximal increase of 14.5-fold was observed 21 h after treatment; Supplementary Fig. 9a ). ABCA1 and ABCG1 , direct targets of LXR/RXR, were also induced immediately after T1317/9cRA treatment ( Supplementary Fig. 9b,c ). MafB deficiency significantly diminished T1317/9cRA-induced AIM mRNA expression to <25% relative to the wild-type control; in contrast, the inducible expression of ABCA1 and ABCG1 was not significantly different between the genotypes ( Supplementary Fig. 9a–c ). Flow cytometry analysis showed that T1317/9cRA treatment increased GFP expression in the Mafb +/− fetal liver macrophages ( Fig. 6b ). Of note, T1317/9cRA treatment barely induced c-Maf expression in wild-type fetal liver-derived macrophages, indicating the more critical contribution of MafB to LXR/RXR-induced AIM expression ( Supplementary Fig. 4b ). We further corroborated these findings by examining human primary macrophages. In human peripheral blood mononuclear cell-derived macrophages, MAFB and ABCG1 expression were indeed activated upon treatment with T1317/9cRA and oxLDL ( Fig. 6c , Supplementary Fig. 11a,b ). Overall, these results indicate that MAFB expression is activated by the ligand-binding heterodimer of LXR/RXR in humans and in mouse primary macrophages. 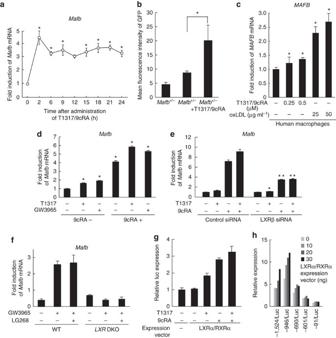Figure 6: MafB is regulated by the LXR/RXR nuclear receptors. (a) Expression ofMafbis induced by LXR and RXR agonists inMafb+/+fetal liver macrophages. Macrophages were incubated with both T1317 (1 μM) and 9cRA (1 μM) for different time periods.MafbmRNA was quantified by qRT–PCR (n=4 for each group). Data were normalized toHprtmRNA; *P<0.05 versus the 0 h time point (Student’st-test). (b) GFP expression inMafb+/+andMafb+/−macrophages treated with or without T1317 (1 μM) and 9cRA (1 μM) for 24 h as determined by flow cytometry analysis (n=3 for each group). *P<0.05 (Student’st-test). (c) Induction ofMAFBexpression by LXR and RXR agonists in human macrophages. Macrophages were incubated with the indicated concentration of oxLDL or the T1317/9cRA mixture. HumanMAFBmRNA was quantified by qRT–PCR (n=4 for each group). Data were then normalized to humanHPRT; *P<0.05 versus vehicle control (Student’st-test). (d,e) qRT–PCR analysis ofMafbmRNA expression. Data were normalized toHprt. (d) RAW264.7 cells were incubated with vehicle, LXR agonists (1 μM T1317 and 5 μM GW3965, either alone or in combination) or 1 μM 9cRA for 24 h (n=4 for each group); *P<0.01 versus vehicle control (Student’st-test). (e) RAW264.7 cells were transfected with either control siRNA or LXRβ siRNA. The cells were then stimulated with T1317 and 9cRA (alone or in combination) for 24 h (n=4 for each group); *P<0.05, **P<0.01 versus matched agonist treatment in cells treated with control siRNA (Student’st-test). (f) WT andLXRDKO peritoneal macrophages were stimulated with GW3965 (1 μM) and LG268 (100 μM) (alone or in combination) for 18 h. Each condition is a pool of three wells from independent experiments. Then, the expression ofMafbmRNA was analyzed by qRT–PCR. Data were normalized to36B4mRNA. The s.d. was representative of the variation in the technical duplicates of the cDNA samples from WT and LXR KO. (g) Relative increase in luciferase activity. The 6.5-kb 5′Mafbpromoter-luciferase constructs were co-transfected with LXRα and RXRα expression vectors (100 ng) in RAW264.7 cells. Then, the cells were treated with T1317 (1 μM) and 9cRA (1 μM) (alone or in combination) for 24 h. Data are from one experiment representative from at least three experiments. Error bars are mean+s.e.m. of duplicate samples. (h) A series of 5′ deletion mutant ofMafbpromoter-luciferase constructs were co-transfected with LXRα and LXRα expression vector with T1317 (1 μM) and 9cRA (1 μM) for 24 h. (a–f) Data are presented as mean+s.e.m. Figure 6: MafB is regulated by the LXR/RXR nuclear receptors. ( a ) Expression of Mafb is induced by LXR and RXR agonists in Mafb +/+ fetal liver macrophages. Macrophages were incubated with both T1317 (1 μM) and 9cRA (1 μM) for different time periods. Mafb mRNA was quantified by qRT–PCR ( n =4 for each group). Data were normalized to Hprt mRNA; * P< 0.05 versus the 0 h time point (Student’s t -test). ( b ) GFP expression in Mafb +/+ and Mafb +/− macrophages treated with or without T1317 (1 μM) and 9cRA (1 μM) for 24 h as determined by flow cytometry analysis ( n =3 for each group). * P< 0.05 (Student’s t -test). ( c ) Induction of MAFB expression by LXR and RXR agonists in human macrophages. Macrophages were incubated with the indicated concentration of oxLDL or the T1317/9cRA mixture. Human MAFB mRNA was quantified by qRT–PCR ( n =4 for each group). Data were then normalized to human HPRT ; * P <0.05 versus vehicle control (Student’s t -test). ( d , e ) qRT–PCR analysis of Mafb mRNA expression. Data were normalized to Hprt . ( d ) RAW264.7 cells were incubated with vehicle, LXR agonists (1 μM T1317 and 5 μM GW3965, either alone or in combination) or 1 μM 9cRA for 24 h (n=4 for each group); * P <0.01 versus vehicle control (Student’s t -test). ( e ) RAW264.7 cells were transfected with either control siRNA or LXRβ siRNA. The cells were then stimulated with T1317 and 9cRA (alone or in combination) for 24 h ( n =4 for each group); * P <0.05, ** P <0.01 versus matched agonist treatment in cells treated with control siRNA (Student’s t -test). ( f ) WT and LXR DKO peritoneal macrophages were stimulated with GW3965 (1 μM) and LG268 (100 μM) (alone or in combination) for 18 h. Each condition is a pool of three wells from independent experiments. Then, the expression of Mafb mRNA was analyzed by qRT–PCR. Data were normalized to 36B4 mRNA. The s.d. was representative of the variation in the technical duplicates of the cDNA samples from WT and LXR KO. ( g ) Relative increase in luciferase activity. The 6.5-kb 5′ Mafb promoter-luciferase constructs were co-transfected with LXRα and RXRα expression vectors (100 ng) in RAW264.7 cells. Then, the cells were treated with T1317 (1 μM) and 9cRA (1 μM) (alone or in combination) for 24 h. Data are from one experiment representative from at least three experiments. Error bars are mean+s.e.m. of duplicate samples. ( h ) A series of 5′ deletion mutant of Mafb promoter-luciferase constructs were co-transfected with LXRα and LXRα expression vector with T1317 (1 μM) and 9cRA (1 μM) for 24 h. ( a – f ) Data are presented as mean+s.e.m. Full size image To thoroughly delineate the regulatory mechanisms of Mafb gene expression by the activated LXR/RXR heterodimer, we examined whether Mafb expression is induced by treatment with LXR/RXR agonists in a macrophage cell line, RAW264.7. Each of two different LXR agonists (T1317 and GW3965) induced Mafb mRNA expression to some extent ( Fig. 6d ). Although treatment with an RXR agonist (9cRA) more significantly induced Mafb mRNA expression, the simultaneous administration of 9cRA with either T1317 or GW3965 increased Mafb induction in an additive manner ( Fig. 6d ). To test whether LXR deficiency leads to a reduction in MafB, we examined the effect of LXRβ loss of function in a RAW264.7 cell line lacking LXRα expression. siRNA against LXRβ successfully reduced LXR β mRNA by 70% ( Supplementary Fig. 11c ). Concomitant with this reduction, ABCA1 mRNA was significantly decreased, whereas the expression of RXR α was barely altered ( Supplementary Fig. 11d,e ). Of note, the T1317/9cRA-stimulated Mafb expression, but not basal Mafb expression, was significantly decreased upon siRNA knockdown of LXRβ, indicating that MafB could not be expressed due to lack of both LXRα and LXRβ ( Fig. 6e ). Furthermore, we analyzed the expression of Mafb in WT and LXR -deficient peritoneal macrophages lacking both LXRα and LXRβ proteins (LXR double knockout (DKO)). Consistent with the siRNA data, the inducible mRNA expression of Mafb and ABCA1 was drastically reduced in LXR DKO macrophages, while that of c-Maf was not significantly different between both genotypes ( Fig. 6f and Supplementary Fig. 11f ). To further elucidate whether LXR/RXR activates Mafb promoter activity, we performed a luciferase reporter assay using the 6.5 kb of sequence upstream of the Mafb promoter region. Although the forcible expression of LXRα/RXRα alone did not necessarily induce Mafb promoter activity, simultaneous treatment with T1317 and 9cRA, together or separately, significantly induced Mafb promoter-driven luciferase activity ( Fig. 6g ). Based on this finding, we next searched for evolutionarily conserved LXR response element (LXRE) sequences within the Mafb gene regulatory region using the UCSC Genome Browser and NUBIscan V2.0, the latter of which is designed to locate putative nuclear receptor transcription factor-binding sites ( http://www.nubiscan.unibas.ch/ ). A series of in silico analyses revealed the presence of a highly conserved LXRE located between −904 and −919 bp of the 5′ Mafb promoter region ( Supplementary Fig. 11g ). To clarify whether this site is important for activating Mafb expression, we performed a luciferase assay using deletion mutants. The −1524/Luc and −946/Luc constructs, which contained LXREs were activated by the LXR/RXR expression vector in a dose-dependent manner. However, the −690, −601 and −91/Luc constructs were not activated by LXR/RXR ( Fig. 6h ). These results suggest that the LXRE between −919 and −904 and LXR/RXR are important for Mafb expression. Overall, these observations indicate that agonist-activated LXR/RXR induces MafB expression, presumably through a conserved LXRE in the upstream regulatory region of the Mafb gene in macrophages. The present study is the first demonstration that MafB deficiency in macrophages leads to accelerated foam-cell apoptosis and that this phenomenon is primarily due to a disruption in the LXR/RXR–AIM regulatory axis. The increased in foam-cell apoptosis resulted in the unexpected amelioration of early atherosclerosis progression. Macrophage apoptosis by itself does not induce the development of atherosclerosis because these cells are cleared by efferocytosis in early lesions. Efferocytosis also induces anti-inflammatory responses during this stage. Therefore, reduced expression of AIM due to Mafb deficiency ameliorates atherosclerosis. By contrast, in advanced lesions, various emerging factors, including oxidative stress, prevent efferocytosis [11] . Owing to this defective efferocytosis in advanced lesions, an increase in macrophage apoptosis leads to necrosis and subsequent induction of the proinflammatory response. Currently, it is difficult to determine the effect of increased apoptosis of Mafb -deficient macrophages on the progression of advanced lesions. Stage-specific conditional deletion of MafB during the process of disease development may provide some insight in future studies. The AIM gene is directly regulated by the LXR/RXR heterodimer [8] , [33] , [34] . This notion was further supported by the identification of a putative functional LXRE located −5,404 bp upstream of the AIM gene [34] . An in vivo experiment showed that LXR α/β-deficient mutant mice exhibit suppressed AIM expression in tissue macrophages [34] . Nonetheless, in other tissues that express low levels of MafB, such as hepatocytes, AIM expression is barely induced by LXR agonist administration despite the abundant expression of LXRα/β and RXR [32] . Given this fact, we assumed that the LXR/RXR-mediated induction of AIM expression might require another factor that is preferentially expressed in macrophages. Our data indicate that LXR/RXR-mediated AIM induction is not detectable in Mafb -deficient macrophages; that is, T1317/9cRA treatment induced AIM expression up to 20-fold in Mafb +/+ macrophages, although the efficacy of this treatment was repressed by less than fourfold in Mafb −/− macrophages. Moreover, in atherosclerotic lesion, expression of AIM was reduced 600-fold in Mafb −/− → LDLR −/− compared with Mafb +/+ → LDLR −/− . Notably, Mafb expression was also induced by T1317/9cRA treatment, while the siRNA-induced downregulation of LXRβ inhibited the inducible expression of Mafb in RAW264.7 cells that lacked LXRα. The LXR DKO also had reduced Mafb mRNA ( Fig. 6e,f ). These observations support a model in which activated LXR/RXR requires Mafb expression for subsequent AIM induction in macrophages. Additionally, Joseph et al . [34] showed that RAW264.7 cells with a native deficiency in LXRα cannot express AIM despite normal LXRβ expression. However, overexpression of LXRα in RAW264.7 cells induced AIM expression. These data indicate that LXRα is required for AIM expression, whereas LXRβ alone is not sufficient. This evidence suggests that LXRα and MafB interact either directly or indirectly; however, further analysis must be performed to confirm this. Taken together, our data indicate that MafB drives the LXR/RXR-induced macrophage-specific transcriptional cascade towards AIM gene expression, potentially through its strong transcriptional activity. Moreover, in human atherosclerotic lesion, both AIM and MAFB were expressed on CD68-positive macrophage region ( Fig. 3g ). In human monocyte-derived macrophage, oxLDL and LXR agonists induced expression of MAFB ( Fig. 6c ). Consequently, MafB may significantly contribute to the magnitude and specificity of AIM expression in foam cells within both mouse and human atherosclerosis. c-Maf, another member of the large Maf family, is also expressed in macrophages and has functions that overlap with those of MafB. Both MafB and c-Maf regulate F4/80 expression in differentiated macrophages [26] , [38] . MafB and c-Maf compound-mutant macrophages cause accelerated proliferation of macrophage-committed progenitors, indicating that these two macrophage-affiliated large Maf factors cooperate to maintain the homeostasis of haematopoietic stem/progenitor fractions [36] . However, the present study showed that AIM expression was barely affected under conditions of c-Maf deficiency ( Supplementary Fig. 4a ). Moreover, c-Maf expression was not induced by pharmacological LXR/RXR activation ( Supplementary Fig. 4b ). Recently, we reported that c-Maf -deficient macrophages fail to form erythroblastic islands, leading to anemia at the embryonic stage due to enucleation defects in erythroblasts. In contrast, the Mafb -deficient embryos do not exhibit a similar anemic phenotype [39] . Overall, these data indicate that MafB and c-Maf play distinct but overlapping roles in macrophages. Further comparative transcriptome analysis using mutant macrophages deficient in each Maf, in combination with chromatin immunoprecipitation coupled with next-generation sequencing (ChIP-seq) analysis, would be particularly useful in further investigations of the shared and/or distinct functions of each large Maf transcription factor in macrophages. Mafb upregulation occurred after ~2 h of agonist treatment ( Fig. 6a ). The mRNA levels of the two representative direct LXR/RXR target genes, ABCA1 and ABCG1 , also exhibited similar responses ( Supplementary Fig. 9b,c ). Both of these gene products mediate cholesterol efflux from macrophages and potentially confer protection against oxysterol-induced toxicity [40] , [41] . The similar response of Mafb (that is, rapid upregulation after LXR/RXR stimulation) implies that the Mafb gene is directly regulated by LXR/RXR nuclear receptors ( Fig. 6a ). This hypohtesis was further supported by a luciferase reporter assay, which demonstrated that LXRα/RXR activated the 6.5-kb Mafb promoter/reporter construct following T1317/9cRA treatment. In fact, we identified a highly conserved LXRE site between −919 and −904 bp of the Mafb promoter region, and we identified two additional conserved distal LXREs at approximately −7,389 to −7,384 and −11,889 to −11,874 bp in the 5′-flanking region of the Mafb gene. The existence of these LXRE clusters suggests that the Mafb gene could be regulated by multiple LXREs ( Supplementary Fig. 11g ). Further analysis to clarify the functional significance of these LXREs would be of particular interest. MafB has a crucial role in the segmentation of rhombomeres 5 and 6 in the hindbrain. Kreisler mutant mice, in which the rhombomere-specific enhancer of the Mafb gene is disrupted by X-ray-induced chromosomal inversion, exhibit abnormal development of the inner ear due to defective segmentation of rhombomere 5 (ref. 42 ). In the rhombomere, the expression of MafB is regulated by a concentration gradient of retinoic acid [43] , [44] , indicating that the Mafb gene is a downstream target of the retinoic acid receptor, which dimerizes with RXR in the hindbrain. Furthermore, MafB is expressed in neural cells, podocytes in the kidney and the lens of the eye [26] , [45] . In all of these systems, retinoic acid plays a key role in promoting correct development [46] . In the current study, we demonstrated that Mafb was regulated by the nuclear receptor LXR/RXR in macrophages. These observations, taken together with our recent data, imply a global epistatic relationship between the nuclear receptor and the Mafb gene. Further exploration of nuclear receptor response elements responsible for Mafb gene expression in each tissue will increase our understanding of the hierarchical regulatory pathway. Animals and fetal liver cell transplantation The Mafb −/− and c-Maf −/− mice used in our experiments were originally generated in a 129/Sv background and were backcrossed to the C57BL/6 strain for more than seven generations. The PCR primers used for genotyping each mutant were described in the previous studies [15] , [26] . LDLR −/− mice (C57BL/6 background) were kindly provided by the Department of Internal Medicine (Metabolism and Endocrinology) of the University of Tsukuba. For haematopoietic cell reconstitution, 1 × 10 7 fetal liver cells were isolated from E14.5–15.5 Mafb +/+ or Mafb −/− (C57BL/6-Ly5.1) embryos (both male and female), and these cells were injected into the tail vein of lethally irradiated (10 Gy) 10- to 12-week-old LDLR −/− (C57BL/6-Ly5.2) male and female mice. The chimerism of the donor cells was determined using the Ly5.1 + /(Ly5.1 + +Ly5.2 + ) cell ratio. Mice with >95% chimerism were used in further experiments. To induce atherosclerosis, the recipient mice were fed an atherogenic diet containing 1.25% cholesterol (Oriental Yeast Co., Ltd.) for 5–12 weeks beginning at 8 weeks post-transplantation. Mice were maintained in specific pathogen-free conditions in a laboratory animal resource center at the University of Tsukuba. All experiments were performed according to the Guide for the Care and Use of Laboratory Animals of the University of Tsukuba. Reagents The agonists used in this study were as follows: T0901317 (T1317, Sigma), GW3965 (Sigma), 9cRA (Sigma), LG100754 (LG754, Tocris Bioscience). rAIM was provided by the Laboratory of Molecular Biomedicine for Pathogenesis of the University of Tokyo. Microarray analysis and quantitative RT-PCR analysis M-CSF-induced fetal liver macrophages from either Mafb +/+ or Mafb −/− E14.5 embryos were prepared as previously described [26] . In brief, single-cell suspensions of fetal liver cells were prepared by mechanical disruption (grinding with a syringe insert against a 70-μm nylon cell strainer; BD Biosciences). Fetal liver cells were resuspended in Dulbecco’s modified Eagle’s medium (DMEM) supplemented with 10% fetal calf serum (heat-inactivated), streptomycin and penicillin (100 units ml −1 ) and M-CSF (R&D Systems, 10 ng ml −1 ) and then seeded onto either tissue culture dish. The culture medium was not changed throughout the experiment. M-CSF (final concentration, 10 ng ml −1 ) was added every day from day 4 onwards. LXR DKO peritoneal macrophages were used for qRT–PCR [34] . Total RNA was prepared using the RNeasy Mini Kit (Qiagen) and expression microarray analysis was performed using purified total RNA. First-strand cDNA was synthesized using the QuantiTect Reverse Transcription Kit (Qiagen). Gene expression profiling was accomplished by hybridization using an Agilent Mouse Oligo Microarray Kit (G412A). The mRNA levels of Mafb , c-Maf , AIM , ABCA1 , ABCG1 , MCP-1 , LXR β, RXR α, human MAFB and human ABCG1 were examined by qRT–PCR using the Thermal Cycler Dice Real Time System (Takara Bio) with SYBR Green PCR master mix (Takara Bio). mRNA abundance was normalized to the mouse Hprt or human HPRT mRNA level. Specific primer sequences are provided in Supplementary Table 1 . Transient transfection assay The 5′-flanking region of the AIM gene was analyzed with the UCSC Genome Browser ( http://genome.ucsc.edu/ ) to predict putative transcription factor-binding sites. The 2.0-kb AIM promoter was PCR-amplified from C57BL/6 mouse genomic DNA using an upstream primer (5′-GGACAATCCACAACAGATACACC-3′) and a downstream primer (5′-GGTTTGAACACTAGAATAAGGAAG-3′). The PCR products were subcloned into a promoter-less luciferase vector (pGL4.10, Promega) to generate the luciferase reporter gene construct (−1993/Luc). The −473/Luc and the −34/Luc plasmids were constructed from −1993/Luc by PCR with upstream primers containing an artificial Kpn I site (500 bp: 5′-CTAG GGTACC CACAGGGATTTGTGGCCATC-3′; 40 bp: 5′-CTAG GGTACC CCTCTATCAGTCCCACCCCCT-3′) and a downstream primer containing an artificial Xho I site (5′-GACT CTCGAG GGTTTGAACACTAGAATAAGGAAG-3′). The −473+mut/Luc plasmid was synthesized using the QuikChange Site-Directed Mutagenesis Kit (Stratagene) using the following primers: 5′-GACCTCCCTTCCTCTGGCCA CAACACCACACAAC CATCTGGCTC-3′ and 5′-GAGCCAGATGGTTGTGTGGT GTTGTGGCCAGAG GAAGGGAGGTC-3′. The italicized sequences indicate the mutated sites. The pGVB2 Mafb promoter constructs, which contain a fragment spanning −6.5 kb to +364 relative to the transcription initiation site and deletion mutants were kindly provided by Dr M. Sakai [47] . The LXRα and RXRα expression vectors were kindly provided by the Department of Internal Medicine (Metabolism and Endocrinology) of the University of Tsukuba. A series of AIM promoter-luciferase constructs were co-transfected with a MafB expression vector [48] into the human lung adenocarcinoma epithelial cell line H441. The Mafb promoter-luciferase constructs were co-transfected with LXRα and RXRα expression vectors into RAW264.7 cells. Transfection was performed using FuGENE6 transfection reagent (Promega), and the cells were harvested 24 h after transfection. For Mafb promoter analysis, the transfected cells were cultured for an additional 24 h in the presence of a mixture of T1317 and 9cRA. The luciferase assay was performed using the Dual-Luciferase Reporter Assay System (Promega) according to the manufacturer’s protocol. Briefly, we transferred up to 20 μl of cell lysate into 100 μl of the Luficerase Assay Reaget ll (LARll). Then samples were placed the tube in the luminometer and initiated reading. Samples were added the 100 μl of Stop & Glo reagent and replaced in the luminometer then initiated reading. Transfection efficiency was routinely normalized to the activity of co-expressed Renilla reniformis luciferase, which was expressed by the pRL-TK (Promega) expression plasmid. Electrophoretic mobility shift assay (EMSA) MafB and mock-control proteins were generated by transiently transfecting 293 T cells with pEFX3-FLAG MafB and pEFX3-FLAG mock, respectively. Nuclear extracts were prepared using the NucBuster Protein Extraction Kit (Novagen). EMSAs and competitive EMSAs were performed using the LightShift Chemiluminescent EMSA Kit (Pierce) according to the manufacturer’s protocol. DNA–nuclear extract binding reactions were performed as follows: 3 μg nuclear extract was pre-incubated for 10 min on ice with 1 × Binding Buffer, 50 ng/μl Poly (dI-dC), 2.5% glycerol, 0.05% NP-40, 50 mM KCl and 5 mM MgCl 2 (from the LightShift Chemiluminescent EMSA Kit). Next, a 200-fold molar excess of cold-competitor double-stranded DNA was added to each reaction, and the reaction mixtures were incubated at room temperature for 5 min. After incubation, biotin-labelled double-stranded DNA probes were added, and the reaction mixture was incubated at room temperature for 20 min. The double-stranded probe and the competitor were generated by annealing the following DNA oligonucleotides (MafB-binding sites are underlined and the mutated sites are italicized): Consensus MARE [12] : 5′-AGCTCGGAAT TGCTGACTCATCA TTACTC-3′ 5′-GAGTAA TGATGAGTCAGCA ATTCCGAGCT-3′ Wild-type AIM MARE: 5′-CTCTGGCCA TGCTGAACTCAGCA CATCTGG-3′ 5′-CCAGATG TGCTGAGTTCAGCA TGGCCAGAG-3′ Mutant competitor: 5′-GACCTCCCTTCCTCTGGCCA CAACACCACACAAC CATCTGGCTC-3′ 5′-GAGCCAGATG GTTGTGTGGTGTTG TGGCCAGAGGAAGGGAGGTC-3′ Atherosclerosis lesion analysis and plasma lipid analysis Lipid deposition was quantified as previously described [8] . Briefly, for en face aorta analyses, mice were killed and the aortic tree was perfused with phosphate-bufferd saline (PBS) followed by 4% paraformaldehyde/PBS. The aorta was dissected en bloc from the root to the iliac bifurcation by removing minor branching arteries and fat tissue. Then, the aortic lumen was opened with a longitudinal incision. After 24 h of fixation in 4% paraformaldehyde, lipids were stained with Oil Red O (Wako), and the stained aortas were then taped to black paper and photographed. The percentage of aortic area stained with Oil Red O was determined using image analysis software (ImageJ and Photoshop). For histological analysis of the aortic roots, PBS-perfused aortas were fixed in 4% paraformaldehyde/PBS for 5 h followed by incubation in 30% sucrose for at least 20 h at 4 °C. Fixed aortas were frozen in OCT embedding medium (Sakura Finetek). Three serial 5-μm sections were cut at 20-μm intervals from the aortic valve area, and the sections were stained with Oil Red O. An equivalent number of aortic valve sites were analyzed in both Mafb +/+ → LDLR −/− and Mafb −/− → LDLR −/− mice. The stained surface area in the sections was quantified using image analysis software (ImageJ and Photoshop). The plasma lipid level was analyzed by a dual enzymatic method using high-performance liquid chromatography (HPLC) (Skylight Biotech Inc.). RNA interference siRNA duplexes of LXRβ were synthesized by Stealth Select RNAi (Invitrogen). Control experiments were performed using Stealth RNAi Negative Control (Invitrogen). The siRNAs were transfected using RNAi Max (Invitrogen) according to the manufacturer’s instructions. Briefly, the opti-MEM containing siRNA and RNAi Max (1:1) were added to the RAW264.7 cells in 1 × 10 5 per well. BLOCK-iT Alexa Fluor Red Fluorescent Oligo (Invitrogen) was used to evaluate the transfection efficiency. siRNA sequences are provided in Supplementary Table 2. Apoptosis assay Macrophages derived from the fetal liver of Mafb +/+ or Mafb −/− littermates were incubated in DMEM culture medium either supplemented with various concentrations of oxLDL or medium without M-CSF. To examine the efficacy of AIM administration or the effect of LXR/RXR activation on apoptosis induction, the macrophages were then cultured with recombinant AIM or a combination of T1317 and 9cRA. Apoptotic cells were detected using the Annexin V-PE Apoptosis Detection Kit (MBL). Briefly, apoptotic cells (1 × 10 5 cells) were collected and added to 5 μl of Annexin V-PE in binding buffer. After incubation for 15 min in the dark, samples were analyzed by flow cytometry without wash step (FACS LSR; BD Biosciences) and CellQuest software. Caspase-3 activity was detected using the Caspase-Glo 3/7 Assay (Promega) according to the manufacturer’s instructions. Briefly, the macrophages (5 × 10 3 cells/well) incubated in a 96-well plate with 100 μl of culture medium were added to 100 μl of Caspase-Glo 3/7 reagent and incubated for 30 min. The luminescence of the samples was measured using the IVIS Spectrum Imaging System (Caliper Life Sciences) and quantified with Living Image software (Caliper Life Sciences). Immunohistochemistry For immunohistochemical analysis of AIM, MafB, GFP, Mac-2, CD31, CD3 and α-actin expression, frozen sections were incubated with a 1:500 dilution of rabbit polyclonal anti-AIM antibody [32] , a 1:1,000 dilution of rabbit anti-MafB (Bethyl), a 1:1,000 dilution of rabbit anti-GFP (MBL), a 1:500 dilution of rat anti-mouse Mac-2 (Cedarlane), a 1:500 dilution of rat anti-mouse CD31 (BD Pharmingen), a 1:500 dilution of rat anti-mouse CD3 (Serotec) or a 1:500 dilution of anti-α-smooth muscle actin (Sigma). For fluorescent staining, a 1:500 dilutions of Alexa Fluor 488-conjugated chicken anti-rat IgG (Molecular Probes), Alexa Fluor 546-conjugated goat anti-rabbit IgG (Molecular Probes), Alexa Fluor 488-conjugated goat anti-rabbit IgG (Molecular Probes) and Cy3-conjugated donkey anti-rat IgG (Jackson ImmunoResearch) secondary antibodies were used. AIM- and Mac-2-stained areas were quantified using Photoshop image analysis software (Adobe Systems). Activated caspase-3 staining was performed using a 1:600 dilution of the anti-cleaved caspase-3 (Asp175) antibody (Cell Signaling). The sections were then visualized with either the Histofine SAB-PO (R) kit or the Histofine SAB-PO (M) kit (Nichirei Bioscience Inc.) according to the manufacturer's instructions. Generation of human macrophages Human monocytes were collected from the peripheral blood of three healthy donors using the RosetteSep Human Monocyte Enrichment Cocktail (StemCell Technologies) and then cultured in RPMI1640 (Sigma) supplemented with 10% fetal bovine serum, 1% penicillin/streptomycin, 1% L -glutamine and 20 ng ml −1 human rM-CSF (R&D Systems) at 37 °C for 5 days. To promote macrophage differentiation, the human monocytes were treated with 10 ng ml −1 IL-10 (R&D Systems) for the next 48 h. To activate the LXRs, the human macrophages were treated with oxLDL or the indicated concentrations of T1317 and 9cRA for another 24 h. The human peripheral blood samples were obtained from donors, who gave informed consent, and with approval from the Ethical Committee of the University of Tsukuba. Chromatin immunoprecipitation and quantitative PCR Fetal liver-derived macrophages were fixed with 1% formaldehyde for 8 min at room temperature. Glycine was added to a final concentration of 0.125 M and the mixture was rotated for an additional 5 min. Cells were washed with ice-cold PBS and resuspended with SDS lysis buffer (10 mM Tris–HCl (pH 8.0), 150 mM NaCl, 1% SDS and 1 mM EDTA). The samples were sonicated to produce chromatin fragments of 200–500 bp and centrifuged at 12,000 g for 10 min. The samples were then diluted in RIPA buffer (10 mM Tris–HCl (pH 7.5), 140 mM NaCl, 1 mM EDTA, 0.5 mM EGTA, 1% Triton X-100, 0.1% SDS, 0.1% Na-deoxycholate and protease inhibitors). After a control aliquot was removed, the samples were incubated with either Dynabeads protein A for immunoprecipitation with rabbit antibodies or Dynabeads anti-mouse IgG antibody for immunoprecipitation with mouse antibodies (Invitrogen), which were preincubated with 1–5 μg of the desired primary antibody. Next, the immunoprecipitated materials were washed and eluted from the beads with elution buffer (25 mM Tris-HCl (pH 7.5), 10 mM EDTA, and 0.5% SDS). After heating at 65 °C overnight, the crosslinks were reversed by incubation in 1.5 mg ml −1 Proteinase K at 55 °C for 2 h. The DNA was purified with a PCR purification kit (Qiagen). The ChIP sample was subjected to quantitative PCR analysis using an ABI7300 system (Perkin Elmer) with SYBR Green Master Mix (Nippon Gene). The PCR signal was normalized relative to that of the input. The sequences of the specific primers targeting the MARE site in the AIM promoter were 5′-GCCACTCAGTCACCTCCCTT-3′ and 5′-CAGGTCCTGTGTGCAGTAGG-3′. FACS analysis of fetal or newborn haematopoietic cells Bone marrow, spleens and peripheral blood cells were isolated from each mouse genotype. Nonspecific binding was blocked by incubation in 5% mouse serum for 15 min, followed by incubation with antibody for 10 min. Phycoerythrin (PE)- or antigen-presenting cell (APC)-conjugated anti-Mac-1, anti-CD8, anti-CD4, anti-B220 (Biolegend) antibodies were used. Flow cytometry analysis was performed with LSR (Becton Dickinson) and the data were analyzed using FlowJo software (Treestar). TUNEL stain Serial 5-μm frozen sections from the proximal aorta were fixed in 4% paraformaldehyde in PBS and treated with 0.2% citric acid. Apoptotic cells were detected by the TUNEL technique using the In Situ Cell Death Detection Kit (Roche Applied Science) and Fast Red TR/Naphthol AS-NX substrate (Sigma). DiI-acetylated LDL and DiI-Ox LDL uptake assays Cells were incubated for 24 h with 5 μg ml −1 1,1′-dioctadecyl-3,3,3′,3′-tetramethylindocarbocyanine (DiI)-labelled acetylated LDL (DiI-AcLDL) or oxidized LDL (DiI-OxLDL; Kalen Biomedical) in DMEM containing 10% ( v / v ) delipidated FCS at 37 °C. Next, cells were released from the tissue culture plate, and DiI-AcLDL or DiI-OxLDL uptake was analyzed by flow cytometry on an LSR flow cytometer (Becton Dickinson). The data were analyzed using FlowJo software (Treestar). ELISA IL-6, IL-10 and IL-12p40 in the culture supernatant were assayed by ELISA using anti-mouse cytokine mAbs as capture Abs, biotin-labelled anti-cytokine mAbs as detection Abs and streptavidin-conjugated alkaline phosphatase (PharMingen) and p-nitrophenylphosphate (Zymed Laboratory) as substrates. Immunohistochemistry of a human section Patients provided informed consent for the analysis of their tissue samples according to the ethics committee of University of Tsukuba Hospital. The atherosclerotic lesion tissue was fixed in 10% formalin and embedded in paraffin blocks, and the most representative block was chosen for each case. Each block was cut into 2-μm-thick serial sections for staining with H&E and immunohistochemistry for CD68, AIM and MAFB. Immunohistochemistry was performed using the EnVision+ dual link (Dako Japan, Tokyo, Japan). The sections were deparaffinized with xylene and rehydrated with ethanol. Antigens were then retrieved by heating at 105 °C for 10 min using an autoclave in TE buffer at pH 9.0 for anti-AIM [32] and MAFB (LifeSpan BioSciences, Inc.). For anti-CD68 (Dako), the section was incubated with proteinase K for 10 min. After blocking endogenous peroxidase activity with a peroxidase-blocking solution (Dako), the sections were incubated with the primary antibodies for CD68 (1:100), AIM (1:500) and MAFB (1:150), diluted in 1% bovine serum albumin in PBS. After washing the sections with PBS, anti-mouse or anti-rabbit HRP-labelled polymer (Dako Japan) was applied at room temperature for 30 min. After washing, the reaction product was visualized with diaminobenzidine (Dako Japan) applied for 5 min. The sections were counterstained with haematoxylin. Statistical analysis The data were recorded as the mean±s.e.m. The statistical significance of the differences among the means of several groups was determined using Student’s t -test. How to cite this article: Hamada, M. et al . MafB promotes atherosclerosis by inhibiting foam-cell apoptosis. Nat. Commun. 5:3147 doi: 10.1038/ncomms4147 (2014). Accession codes: Microarray data have been deposited in the National Center for Biotechnology Information Gene Expression Omnibus under accession code GSE20419 .